Spin wave-assisted reduction in switching field of highly coercive iron-platinum magnets Recent rapid progress in spintronic and magnetic storage nanodevices has required nanomagnets to balance competing goals for high coercive field and low switching field. However, a decisive route for highly efficient magnetization switching has not been established yet. Here we propose a novel switching method using a spin wave of magnetic structures twisted in a nanometre scale. We have experimentally demonstrated extremely low field-magnetization switching in a highly coercive FePt by using a spin wave excited in a soft magnetic permalloy (Ni 81 Fe 19 ), where permalloy is exchange-coupled to FePt through the interface. We can tune the switching field by varying the magnitude and frequency of the radio frequency magnetic field, and a significant decrease in switching field by one order of magnitude is achieved under the optimum conditions. The spin wave-assisted magnetization switching is a promising technique for ultralow-energy magnetization manipulation. A route simultaneously achieving competing goals for good thermal stability of magnetization (high coercive field H c ) and low switching field H sw is indispensable for the further development of spintronic and magnetic storage nanodevices [1] . Energy-assisted switching [2] , [3] , [4] , [5] , [6] , [7] , [8] , [9] , [10] , [11] , [12] , spin-transfer switching [13] , [14] and voltage-induced H c modulation [15] are examined to overcome this predicament. One of the energy-assisted switching methods is microwave-assisted magnetization reversal (MAMR), which is considered to be a promising recording method for future ultrahigh density magnetic storage [2] , [3] , [4] , [5] , [6] , [7] , [8] , [9] . It applies a radio-frequency (rf) magnetic field H rf to a highly coercive magnet to obtain induction of uniform magnetization precession to reduce H sw . However, MAMR has an inherent undesirable characteristic. The frequency of H rf is around the ferromagnetic resonance (FMR) frequency f FMR , which is of the order of 100 GHz for a highly coercive magnet. This is a serious obstacle for practical applications. Indeed, although several papers [3] , [4] , [5] reported H sw reduction at single-digit gigahertz frequencies using soft magnetic materials such as a Ni–Fe alloy with f FMR <10 GHz, a high excitation frequency >10 GHz was required in the case of a highly coercive magnet with f FMR >10 GHz [7] , [8] . There are no reports of clear H sw reduction for a highly coercive magnet at single-digit gigahertz frequencies. Thus, another way of reducing H sw while maintaining high H c is desired. The concept of magnetization switching presented here is based on the utilization of spin wave modes in a soft magnet to switch the magnetization in a hard magnet. A similar method has been theoretically proposed by Li et al. [16] and Fal et al. [17] However, there has been no experimental demonstration to date as far as we are aware. Here we show the significant reduction in H sw of highly coercive FePt due to the spin wave excitation. Magnetic structure and FMR We combined a hard magnetic FePt layer with a soft magnetic permalloy (Fe 19 Ni 81 ; Py) layer, as schematically illustrated in Fig. 1a . In this FePt/Py bilayer, FePt has an uniaxial easy magnetization axis along the in-plane [001] direction. The magnetic moments in Py are spatially twisted after the magnetic field H has been applied in the opposite direction to the magnetic moments in FePt [18] . The Py layer thickness t Py was varied in the range from 40 to 120 nm, whereas the FePt layer thickness was fixed at 10 nm. The full magnetization loop of an FePt/Py bilayer with t Py =100 nm ( Fig. 1b ) shows two steep decreases in magnetization. The first steep decrease at around H =−100 Oe corresponds to the twist of magnetic moments in Py. The second steep decrease at around H =−1,600 Oe means that the bilayer’s magnetization has switched. The minor loop is superimposed on the full loop. After all the magnetizations has been saturated in the positive direction at H =50 kOe, H was swept to −1,400 Oe (magenta circles). Then, H was returned to zero (cyan circles). The minor loop is completely reversible without any hysteresis. This behaviour is well known as spring-back [19] , indicating that FePt and Py are exchange-coupled through the interface and that the magnetic moments in Py are spatially twisted by applying H . 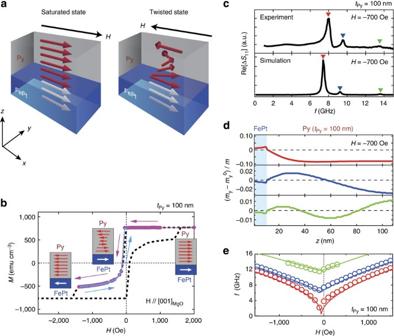Figure 1: Magnetization loops and FMR for an FePt/Py bilayer. (a) Illustrations of magnetic structures in an FePt/Py bilayer. The left (right) panel depicts the direction of magnetic moments in the saturated (twisted) state together with the coordinate axes. Magnetic fieldHwas applied along the in-plane [001] direction of the MgO (110) substrate, which corresponds to the easy magnetization direction of FePt. (b) Magnetization full loop (dashed line) and minor loop for the bilayer with the Py layer thicknesstPyof 100 nm. For the minor loop measurements,H=50 kOe was first applied to saturate all the magnetizations in the positive direction. Then,Hwas swept to −1,400 Oe (magenta circles) and back to zero (cyan circles). (c) FMR spectra oftPy=100 nm for experiment (upper panel) and simulation (lower panel) atH=−700 Oe. The triangles indicate the resonant frequencies. (d) Snapshots of the deviation of magnetic moments from the equilibrium position in theydirectionmy–my0. The red, blue and green curves correspond to the first, second and third FMR peaks, respectively. These excitation modes are the PSSW modes withn=0 (red),n=1 (blue) andn=2 (green), wherenis the number of nodes. The interface between FePt and Py is located atz=10 nm. (e) Experimentally obtained resonant frequencies ofn=0 (red),n=1 (blue) andn=2 (green) plotted as a function ofHfortPy=100 nm (open circles). The simulated resonant frequencies are also shown by solid lines. Figure 1: Magnetization loops and FMR for an FePt/Py bilayer. ( a ) Illustrations of magnetic structures in an FePt/Py bilayer. The left (right) panel depicts the direction of magnetic moments in the saturated (twisted) state together with the coordinate axes. Magnetic field H was applied along the in-plane [001] direction of the MgO (110) substrate, which corresponds to the easy magnetization direction of FePt. ( b ) Magnetization full loop (dashed line) and minor loop for the bilayer with the Py layer thickness t Py of 100 nm. For the minor loop measurements, H =50 kOe was first applied to saturate all the magnetizations in the positive direction. Then, H was swept to −1,400 Oe (magenta circles) and back to zero (cyan circles). ( c ) FMR spectra of t Py =100 nm for experiment (upper panel) and simulation (lower panel) at H =−700 Oe. The triangles indicate the resonant frequencies. ( d ) Snapshots of the deviation of magnetic moments from the equilibrium position in the y direction m y – m y 0 . The red, blue and green curves correspond to the first, second and third FMR peaks, respectively. These excitation modes are the PSSW modes with n =0 (red), n =1 (blue) and n =2 (green), where n is the number of nodes. The interface between FePt and Py is located at z =10 nm. ( e ) Experimentally obtained resonant frequencies of n =0 (red), n =1 (blue) and n =2 (green) plotted as a function of H for t Py =100 nm (open circles). The simulated resonant frequencies are also shown by solid lines. Full size image We measured the FMR spectra of the FePt/Py bilayers using a coplanar waveguide (CPW) and a vector network analyser [20] , [21] (see Methods). Figure 1c shows the FMR spectrum for t Py =100 nm at H =−700 Oe under the application of H rf =6 Oe. We observed three resonant peaks at the frequencies f =8.0, 9.5 and 13.5 GHz, as indicated by red, blue and green triangles, respectively. The shape of the experimental FMR spectrum is well reproduced by the simulation (for more details of experimental FMR spectra, see Supplementary Fig. S1 ). To classify the excited magnetization dynamics at each resonance, we plotted snapshots of the deviation of magnetic moments from the equilibrium position in Fig. 1d . The red, blue and green curves correspond to the first, second and third FMR peaks, respectively. These excitation modes are known as the perpendicular standing spin wave (PSSW) modes [22] with n nodes. Figure 1e shows the experimental results for the H dependence of resonant frequencies (open circles) together with the simulated results (solid lines). The simulated results were obtained using the calculation method reported by Livesey et al. [23] (for more details, see Methods). We successfully observed the higher-order PSSW modes, which have never been reported for previous experimental studies [24] , [25] , [26] , and the frequencies of all modes agree well with the simulation. The present results are also in good agreement with the simulation reported by Fal et al. [17] Looking at Fig. 1d carefully, one can see that the dynamics of magnetic moments in FePt are also induced by PSSW. In other words, depinning occurs in FePt due to the excitation of PSSW in Py. This leads us to the idea that high H rf enhances the amplitude of PSSW and should reduce H sw of the FePt/Py bilayer. Spin wave-assisted magnetization switching We microfabricated rectangular FePt/Py bilayer elements on the signal line of a CPW ( Fig. 2a ) to study the H sw reduction by PSSW. The device resistance R depends on the direction of magnetic moments in the FePt/Py bilayer owing to the anisotropic magnetoresistance effect [27] , [28] . 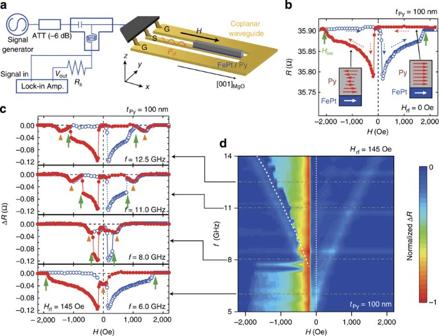Figure 2: Spin wave-assisted magnetization switching. (a) Schematic illustration of the device structure and measurement setup. The rf power was applied from a signal generator through the rf port of a bias-Tee. The device resistanceRas a function ofHwas measured using a lock-in amplifier.Rsis a reference resistance of 1 kΩ. The FePt/Py was designed to be rectangular, 2 × 50 μm2. (b)R–Hcurve fortPy=100 nm without the rf magnetic fieldHrf. The green arrows denote the switching fieldsHsw. (c) ΔR–Hcurves fortPy=100 nm under the application ofHrf=145 Oe, where ΔRis the resistance change from the baseline resistance. The frequenciesfofHrfwere 12.5, 11.0, 8.0 and 6.0 GHz. The small dips in ΔRdue to the excitation of PSSW are indicated by orange triangles. (d) Two-dimensional map of normalized ΔRas functions ofHandffortPy=100 nm.Hwas swept from positive to negative. The white dotted line denotes the resonant frequency of PSSW withn=0 in the twisted state of the microfabricated sample. Figure 2b shows the R – H curve for t Py =100 nm without H rf being applied. When H was swept from positive to negative (denoted by red circles), R showed an abrupt decrease at H =−175 Oe, reflecting the twist of magnetic moments in Py. R returned to the baseline resistance R B at H = H sw =−2,050 Oe (green arrows), where the magnetic moments of the bilayer were switched. Figure 2c displays Δ R – H curves for t Py =100 nm with H rf =145 Oe, where Δ R is defined as R – R B . No remarkable changes in H sw were observed for f =6.0 GHz. However, the application of H rf with f =8.0 GHz reduced H sw to 325 Oe. As f was increased from 8.0 to 12.5 GHz, H sw monotonically increased. Small dips in Δ R appeared in the saturated state, which are indicated by orange triangles. A two-dimensional map of normalized Δ R as functions of H and f is shown in Fig. 2d . H was swept from positive to negative. The H sw reduction was obtained in the wide range of f from 8 to 14 GHz. The small dip in Δ R has the same dispersion as that of PSSW in the saturated state. To understand what determined the value of H sw at each f , we overlapped the resonant frequency of PSSW with n =0 in the twisted state of the microfabricated sample (white dotted line). Note that the frequency dependence of H sw qualitatively followed that of the resonant magnetic field of PSSW H PSSW , indicating that magnetization switching was induced by PSSW as we expected. Figure 2: Spin wave-assisted magnetization switching. ( a ) Schematic illustration of the device structure and measurement setup. The rf power was applied from a signal generator through the rf port of a bias-Tee. The device resistance R as a function of H was measured using a lock-in amplifier. R s is a reference resistance of 1 kΩ. The FePt/Py was designed to be rectangular, 2 × 50 μm 2 . ( b ) R – H curve for t Py =100 nm without the rf magnetic field H rf . The green arrows denote the switching fields H sw . ( c ) Δ R – H curves for t Py =100 nm under the application of H rf =145 Oe, where Δ R is the resistance change from the baseline resistance. The frequencies f of H rf were 12.5, 11.0, 8.0 and 6.0 GHz. The small dips in Δ R due to the excitation of PSSW are indicated by orange triangles. ( d ) Two-dimensional map of normalized Δ R as functions of H and f for t Py =100 nm. H was swept from positive to negative. The white dotted line denotes the resonant frequency of PSSW with n =0 in the twisted state of the microfabricated sample. 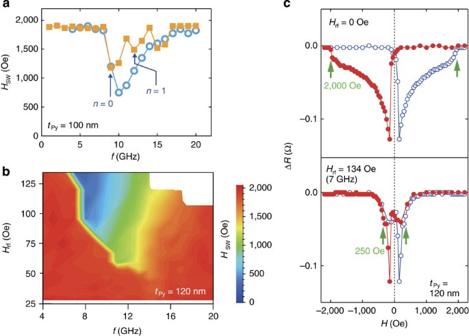Figure 3: Optimum conditions ofHrfandfforHswreduction. (a)Hswas a function offfortPy=100 nm (circles), where the value ofHrfwas set to 91 Oe. SimulatedHswas a function offis also shown by closed squares. (b) Two-dimensional map ofHswas functions ofHrfandffortPy=120 nm. (c) ΔR–Hcurves fortPy=120 nm withHrf=0 Oe (top panel) and 134 Oe (bottom panel). The frequency ofHrfwas 7 GHz. Full size image Figure 3a shows the f dependence of H sw for t Py =100 nm obtained experimentally (circles) and numerically (squares). The experimental results qualitatively coincide with the simulation. The largest reduction in H sw was achieved at f =10 GHz in the experiment, whereas the simulation showed the largest H sw reduction at around f =9 GHz. The simulated result has two local minima of H sw . Analysing the PSSW mode contributing to the magnetization switching, we found that these two local minima originated from the PSSW modes with different n . Because the experiments were performed at room temperature, these two local minima of H sw were smeared out. For both experiment and simulation, H rf with low f is ineffective for H sw reduction because the resonant magnetic field at such low f is so low that it cannot twist the magnetic moments enough to reduce H sw at H rf =91 Oe. Spin wave-assisted magnetization switching was also attempted for the FePt/Py bilayer with t Py =40 nm. We did not observe any H sw reduction even when H rf =113 Oe was applied (see Supplementary Fig. S2 ). This result provides two important facts: the excitation of the FMR mode in FePt does not contribute to the H sw reduction (see Supplementary Fig. S3 ), and a thin Py layer is not effective for H sw reduction. Figure 3: Optimum conditions of H rf and f for H sw reduction. ( a ) H sw as a function of f for t Py =100 nm (circles), where the value of H rf was set to 91 Oe. Simulated H sw as a function of f is also shown by closed squares. ( b ) Two-dimensional map of H sw as functions of H rf and f for t Py =120 nm. ( c ) Δ R – H curves for t Py =120 nm with H rf =0 Oe (top panel) and 134 Oe (bottom panel). The frequency of H rf was 7 GHz. Full size image Figure 3b shows H sw as functions of f and H rf for the FePt/Py bilayer with t Py =120 nm. The frequency giving the lowest H sw decreased as H rf was increased. We successfully achieved the largest reduction in H sw from 2,000 to 250 Oe at f =7 GHz and H rf =134 Oe ( Fig. 3c ). Let us introduce the rate of H sw reduction defined as , where H sw 0 is H sw without H rf . According to the MAMR calculation reported by Zhu et al. [6] , H sw 0 =5.3 H rf and H sw =1.5 H rf . Consequently, δH sw for MAMR is about 0.27, which is twice as high as that of spin wave-assisted magnetization switching, δH sw =0.13. We examined the nonlinear magnetization dynamics in the FePt/Py bilayer because large H rf was applied for spin wave-assisted switching. FMR spectra for the microfabricated device were also measured under the application of large H rf (see Supplementary Fig. S4 ), and clear resonant peaks were observed as in the case of small H rf . The linewidth of resonant peaks became broadened and the asymmetric peak shape was observed for large H rf , which may be related to the nonlinear magnetization dynamics. However, more pronounced nonlinear effects, such as remarkable nonlinear frequency shift, were not observed. This is different from nonlinear magnetization dynamics observed in spin torque oscillators [29] , where spatially uniform magnetization precession is induced by spin-polarized electric current. The precession frequency of a spin torque oscillator depends on the precession angle because the change in the precession angle leads to the large change in the effective field. On the other hand, the PSSW mode observed in this study is spatially non-uniform magnetization dynamics, and its precession frequency is mainly determined by the exchange field. The exchange field does not depend on the precession angle. Thus, the absence of the remarkable nonlinear frequency shift for the present devices is attributable to the less dependence of effective field on the precession angle. An important point is that the PSSW modes were well defined even under the large H rf application. To understand the magnetization dynamics during switching, the time evolution of magnetization switching behaviour was simulated numerically. 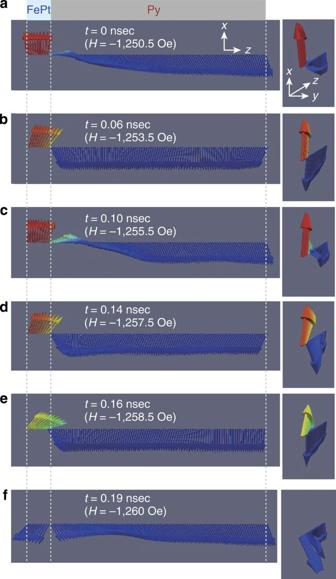Figure 4: Time evolution of magnetization switching behaviour. Simulated magnetic structures in thex–zplane (left panels) and thex–yplane (right panels), whereHrf=90 Oe withf=10 GHz was applied.Hwas swept from 0 to −1,500 Oe, and the magnetization switching occurs in the range fromH=−1,250.5 Oe (a) toH=−1,260 Oe (f). (a–f) The time-evolved snapshots of magnetic structures during the magnetization switching. Figure 4 shows the snapshots of simulated magnetic structures during magnetization switching under the application of H rf =90 Oe with f =10 GHz (for more details, see Supplementary Movie 1 and Supplementary Table 1 ), where H was swept from 0 to −1,500 Oe, and the magnetization switching occurs in the H range from −1,250.5 ( Fig. 4a ) to −1,260 Oe ( Fig. 4f ). The amplitude of the PSSW mode in Py is resonantly enhanced, which increases the precessional amplitude of FePt at the interface, and all the magnetic moments are finally switched. The PSSW mode with n =0 largely contributes to the H sw reduction compared with the other modes ( n =1 and 2). According to the simulated result ( Fig. 3a ), n =1 could also reduce H sw at the resonant frequency, although the H sw reduction is not so significant and is smeared out in the experiment. A reason for the large H sw reduction by n =0 is the larger precession amplitude for n =0 than those for n =1 and 2 (see Fig. 1d and Supplementary Fig. S5 ). As shown in Fig. 4 , the large amplitude magnetization precession in Py induces the large amplitude magnetization precession in FePt, which effectively switches the magnetization of FePt. Figure 4: Time evolution of magnetization switching behaviour. Simulated magnetic structures in the x – z plane (left panels) and the x – y plane (right panels), where H rf =90 Oe with f =10 GHz was applied. H was swept from 0 to −1,500 Oe, and the magnetization switching occurs in the range from H =−1,250.5 Oe ( a ) to H =−1,260 Oe ( f ). ( a – f ) The time-evolved snapshots of magnetic structures during the magnetization switching. Full size image The numerical simulation indicates that the spin wave excitation leads to the magnetization switching in FePt. However, one might think that in the experiment, H sw is not the real switching field of FePt, but the depinning field in FePt layer because depinning occurs in FePt under the large H rf application. We confirmed that H sw corresponded to the real switching field of FePt from the anisotropic magnetoresistance curves measured using different sequences of magnetic field sweep (see Supplementary Fig. S6 ). One might also suspect that the origin of H sw reduction is the temperature rise due to the application of H rf , that is, Joule heating by alternating current. However, this idea can be eliminated because R B , which is a function of the device temperature, did not show any dependence on f (see Supplementary Fig. S7 ). The large H sw reduction by spin wave excitation was also confirmed for the other devices (see Supplementary Table S2 ), indicating that the error in the rate of H sw reduction is small. Because our results simultaneously achieved the competing goals of both high H c and low H sw , spin wave-assisted magnetization switching provides a new nanotechnology for information writing in a wide range of spintronic and magnetic storage applications. Thin film preparation Thin films were prepared on a MgO (110) single-crystal substrate. The stacking of the thin films was MgO (110) substrate/Fe (1 nm)/Au (40 nm)/FePt (10 nm)/Py ( t Py )/Au (3 nm). The layers from Fe to FePt were deposited by using an ultrahigh vacuum (UHV) magnetron sputtering system (ULVAC, Inc.) equipped with high-purity targets of Fe (99.99%), Pt (99.99%) and Au (99.9%). The base pressure of the UHV magnetron sputtering system was below 2 × 10 −7 Pa. A 1-nm thick Fe seed layer and a 40-nm thick Au buffer layer were deposited at ambient temperature. Subsequently, a 10-nm thick FePt layer was deposited on the Au buffer layer after the substrate temperature was set at 450 °C. Then, the film was transferred from the UHV magnetron sputtering chamber to an ion beam sputtering (IBS) system. In the IBS chamber, a Py layer followed by a 3-nm thick Au capping layer was deposited on the FePt layer at ambient temperature. The compositions of FePt and Py were determined to be Fe 48 Pt 52 and Ni 81 Fe 19 , respectively, by electron probe X-ray microanalysis. The epitaxial growth of Au, FePt and Py layers with the (110) preferential crystallographic orientation was confirmed by X-ray diffraction. The X-ray diffraction patterns also indicated the formation of the L 1 0 ordered structure in the FePt layer. The magnetization loops of the thin films were measured at 295 K using a superconducting quantum interference device magnetometer. FMR measurement The FMR measurement was carried out at room temperature using a CPW and a vector network analyser. A thin film with a FePt/Py bilayer was put onto the CPW consisting of Cr/Au layers, and the CPW was connected to the rf circuit employing a two-terminal rf probe. The rf power P rf of 0 dBm was applied to the signal line, which induced a transverse rf magnetic field of H rf ~6 Oe, and the change in the reflected signal was detected with the vector network analyser. The value of S 11 is defined as the ratio of the reflected voltage to the input voltage. The frequency dependence of S 11 was measured under the application of H , which was applied along the in-plane easy magnetization direction. Device fabrication and electrical measurement Rectangular-shaped FePt/Py elements were prepared by using a conventional microfabrication process. First, a negative-type electron beam (EB) resist was spin-coated onto the thin film and patterned into the shape of the CPW by EB lithography (ELS-7500; Elionix Inc.). The width and length of the signal line of CPW were 4 and 50 μm, respectively. After exposure of the EB resist followed by development, the thin film was milled by argon ions through the resist mask. The EB resist was then spin-coated onto the CPW-shaped film and patterned into a rectangular shape with the size of 2 × 50 μm 2 , which was located on top of the signal line of the CPW-shaped film. The CPW-shaped film was again milled by argon ions. The ion milling was stopped at the top of the Au buffer layer, which was monitored by secondary ion mass spectroscopy. Finally, the Au buffer layer remained as the signal and ground lines of the CPW, and the rectangular FePt/Py element was prepared on the signal line. This rectangular shape induces the shape anisotropy of Py. Because the long axis of rectangle is the same as the in-plane [001] direction of the FePt layer, both uniaxial easy magnetization axes of FePt and Py are in the same direction. The microfabricated device was connected to the rf-compatible circuit via a two-terminal rf probe, and P rf was applied from a signal generator through the rf port of a bias-Tee after −6 dB attenuation. The application of P rf induced H rf in the y–z plane of the FePt/Py element. The device resistance was simultaneously measured using a lock-in amplifier. Numerical simulation Numerical simulation was carried out by solving the Landau–Lifshitz–Gilbert (LLG) equation by using the conventional fourth-order Runge–Kutta algorithm. The effective magnetic field in the LLG equation is the vector sum of the anisotropy field, magnetostatic field, exchange field, H , and H rf . In the present numerical study, we considered an exchange-coupled FePt/Py bilayer of infinite size in the film plane. The thicknesses of FePt and Py were fixed at 10 and 98 nm, respectively. The film was discretized into 1-nm thick infinite plates, and each plate was assumed to have a uniform magnetization vector. The saturation magnetizations of FePt and Py were determined to be 1000 and 800 emu cm −3 , respectively, from the magnetization measurement. The inter- and intra-layer exchange constants of FePt/Py, A int , A FePt and A Py , were chosen to be 1.0 × 10 −7 , 1.0 × 10 −6 and 1.3 × 10 −6 erg cm −1 , respectively, so as to reproduce the experimental magnetization loop. The small value of A int results from the slight oxidation and/or the contamination on the FePt surface during the sample transfer from the UHV magnetron sputtering system to the IBS system with breaking the vacuum. The uniaxial anisotropy constant of FePt K FePt was assumed to be 3.3 × 10 6 erg cm −3 , which was determined from the magnetic field required to switch FePt in the lithographically patterned device (see Fig. 2b ), whereas K Py was set to 1.0 × 10 3 erg cm −3 . One may consider that K FePt =3.3 × 10 6 erg cm −3 is small. The one-dimensional model often leads to the underestimation of K FePt to reproduce H sw because in experiment H sw is generally much smaller than the anisotropy field. The experimental value of K FePt was about 2.5 × 10 7 erg cm −3 . The Gilbert damping constants for Py and FePt were 0.008 and 0.02, respectively. To evaluate the H sw reduction under the H rf application, we set H rf to 90 Oe. When H sw as a function of f was evaluated, the magnetization was initially magnetized along + x direction. The magnetization was relaxed for 10 ns under H rf applied along the y axis. The magnetization curve under the H rf application was then calculated sweeping the dc magnetic field along the x direction. The field sweep velocity was 50 Oe ns −1 . H sw was defined as the magnetic field at which the magnetization of the FePt layer became zero. To obtain the f dependence of H sw , f was varied in the range from 1 to 20 GHz. Using the same parameters as those for the magnetization switching simulation, we calculated the stable magnetic structure at each H by solving the LLG equation. For these stable magnetic structures, we solved the eigenvalue equations corresponding to the linear response to the small H rf and obtained the resonant frequencies. To construct the eigenvalue equations, we employed the local rotated frame where the coordinates are rotated about the z axis such that the new x axis points in the same direction as the local magnetization vectors. How to cite this article: Seki, T. et al. Spin wave-assisted reduction in switching field of highly coercive FePt magnets. Nat. Commun. 4:1726 doi: 10.1038/ncomms2737 (2013).